Rotational dynamics of cargos at pauses during axonal transport Direct visualization of axonal transport in live neurons is essential for our understanding of the neuronal functions and the working mechanisms of microtubule-based motor proteins. Here we use the high-speed single particle orientation and rotational tracking technique to directly visualize the rotational dynamics of cargos in both active directional transport and pausing stages of axonal transport, with a temporal resolution of 2 ms. Both long and short pauses are imaged, and the correlations between the pause duration, the rotational behaviour of the cargo at the pause, and the moving direction after the pause are established. Furthermore, the rotational dynamics leading to switching tracks are visualized in detail. These first-time observations of cargo's rotational dynamics provide new insights on how kinesin and dynein motors take the cargo through the alternating stages of active directional transport and pause. Axonal transport of proteins and materials inside the cytoplasm of the slender axon is essential for a neuron's growth and function. For example, proteins manufactured by ribosomes need to be delivered anterogradely from the cell body and distributed along the axon, whereas extracellular materials internalized through endocytosis at the distant axon outposts are moved retrogradely towards the cell body for degradation. Dysfunction of axonal transport may lead to serious neuronal disorders such as the Alzheimer's disease, which is related to the abnormal depolymerization of microtubules inside the axon [1] . Besides its physiological significance, axonal transport is a model system for studying the mechanisms of intracellular transport by motor proteins in mammalian cells. The microtubule arrays located inside the axon have the same polarity, with the minus end facing the cell body. The motor proteins kinesin and dynein transport cargos in the anterograde and retrograde directions, respectively, by 'walking' on the microtubule arrays [2] . The underlying mechanism of axonal transport has been studied intensively for several decades [3] , [4] , [5] , [6] , [7] , [8] . Cargos are moved between the cell body and the synapse via fast and slow axonal transport. It has been found that membranous cargos are generally fast transport components [8] , while cytoskeletal structures [9] , [10] , [11] and non-membrane-bound proteins [6] , [12] are slow transport components. Both slow- and fast-transport cargos move at comparable speeds when they are actually moving, and the transport efficiency is determined mainly by the fraction of time they spend in moving [8] . Cargos pause much more frequently and for longer durations in the slow transport than in the fast transport. The 'Stop and Go' model suggests that the pauses are caused by the varying affinities between the cargo and motor proteins in slow axonal transport [5] , [13] , [14] . When the coupling between the cargo and the motor proteins is deficient, the cargo can fall off the microtubule to pause the transport. Another hypothesis suggests that the pauses are a result of tug-of-war among motor proteins of opposing directionality [15] , [16] , [17] . Understanding the mechanism of axonal transport relies on our knowledge on how the two motor proteins of opposing directionality move a cargo. The tug-of-war model supports the idea that the two motor proteins compete with each other to move the cargo in their desired direction [16] , [17] , [18] , [19] . On the contrary, the coordination model suggests that the two types of motor proteins are coordinated by certain molecular signals so that only one is activated while the other is deactivated during transport [20] , [21] , [22] , [23] , [24] , and a coordination complex might exist to regulate the motors [25] , [26] , although this coordination complex was proved unnecessary to explain the bidirectional cargo transport [17] . It was also proposed that the two models coexist in the microtubule-based transport, while tug-of-war can be deemed as one mechanism of 'coordination' [15] . In this model, multiple kinesin and dynein motors bind to the cargo at the same time, and communication and coordination are achieved through the engaging and disengaging of motor proteins under competing pulling forces; the moving direction of the cargo is directly decided by the number of motors that engage in the tug-of-war [27] , [28] , [29] . Recently, Schuster et al . [30] showed that the change in the transport direction is influenced by the binding and unbinding of dynein motors to the organelles, and Kunwar et al . [31] used the theoretical 'mean field' model to show that an additional level of regulation is necessary to combine with 'tugs-of-war' to explain the in vivo transport data, while the 'sharp maxima approximation' approach was also shown to be able to quantitatively describe the stochastic dynamics of the tug-of-war model [19] . Direct visualization of the transport events in living neurons has led to the current understanding of the mechanism of axonal transport. For example, the axonal transport of organelles has been visualized in real-time using fluorescence-based techniques [9] , [12] , [32] . Pseudo total internal reflection fluorescence microscopy has been applied in tracking the axonal transport of nerve growth factor-modified quantum dots incorporated in endosomes [33] . However, the mechanics of the pauses in the transit of cargos are still largely unknown, mainly because of the limitations of the molecular or nanoparticle probes used in the previous studies. No orientation or rotational information of the cargo at the pauses was disclosed. The cargo's rotational dynamics at the pauses is the direct consequence of motor protein competition and regulation and thus is essential to fully understand axonal transport. In all of the previous reports, the cargo itself or the labels on the cargo gave constant image contrasts at a seemingly fixed location during a pause. It was unclear whether the cargo was completely fixed in space with no motion at all or it was still rotating at various speeds. Recently, we introduced the single particle orientation and rotational tracking (SPORT) technique [34] , [35] , [36] to follow the rotational motion of plasmonic gold nanorods [37] under a differential interference contrast (DIC) microscope. Working in the principle of interferometry [38] , a DIC microscope generates disproportionate bright and dark interference patterns for gold nanorods in different orientations. The relative bright and dark intensities are independent measures of the effective projections of the nanorods onto the two polarization axes, from which the gold nanorod's 3D orientation can be resolved in each DIC image. By measuring the bright and dark DIC intensities of the gold nanorod continuously, it becomes possible to dynamically track the nanorod's orientation and rotational patterns. Using the SPORT technique with an electron-multiplying charge-coupled device running at a temporal resolution of 30 ms, we observed that a cargo tends to keep the same orientation relative to the microtubule tracks during the active transport in living cells [34] . In the current study, we acquired for the first time the orientation and rotational information of the cargo during both the moving (directional transport) and pausing stages of axonal transport at a high temporal resolution of 2 ms. This high temporal resolution was achieved by using a scientific complementary metal-oxide-semiconductor (CMOS) camera when limiting the region of interest to a narrow stripe that was aligned with the axon where the transport events occurred. Such a high temporal resolution is necessary to resolve the motions of cargo in unprecedented detail and answer some of the outstanding questions on the mechanism of axonal transport. Rotation of endocytic vesicles reported by gold nanorods The gold nanorods with an average size of 25×73 nm were used as orientation and rotational nanoprobes. Supplementary Fig. S1 shows a set of DIC images for a gold nanorod that was immobilized on a glass slide and rotated to different orientations with an interval of 10°. The gold nanorods were surface-modified with transferrin (a glycoprotein used as a drug delivery agent [39] ) through a polyethylene glycol (PEG) linker to facilitate receptor-mediated endocytosis. After endocytosis, these nanorods were transported inside the endocytic vesicles by motor proteins along the cytoskeletal tracks. Some of the nanorod-containing vesicles were found to be transported in the axons anterogradely or retrogradely. For a gold nanorod to report the vesicle's rotational motion accurately, the nanorod is required to be stationary with respect to the vesicle on the time scale of the transport events. This requirement is generally met when a single nanorod is contained within the lipid membranes of a small endocytic vesicle, which has a size comparable to the size of the nanorod, and is bound to the transferrin receptors imbedded in the lipid membrane. Supplementary Fig. S2 is a transmission electron micrograph showing gold nanorod-containing vesicles in a PC12 cell. However, after the endocytic vesicle fuses with an early or late endosome, there is more room for the nanorod to rotate randomly, losing its ability to report the rotational motions of the vesicles. An example that the nanorods cannot be used as the orientation and rotational reporter is provided in Supplementary Movie 1 . Apparently, the two nanorods in this movie were transported together inside the same endosome, and they were free to perform rotational and translational Brownian motions. The qualification of each individual nanorod as orientation and rotational reporter must be verified by checking whether the nanorod maintained a constant DIC image pattern during the undisrupted linear transport. This criterion is based on the fact that cytoplasmic microtubules in mammalian cells, including PC12 cells, are composed of 13 linear protofilaments [40] , and that kinesin and dynein motor proteins pull the cargos along the linear protofilament tracks if there are no interruptions (for example, obstacles, dissociation of motors from the tracks or degraded microtubules) to the transport [41] , [42] . A constant DIC image pattern during the linear transport events suggests that the nanorod and its lipid vesicle maintain their orientation relative to one another and to the microtubule tracks as we have reported previously [34] . The restriction on the cargo's rotational motion during the directional transport is believed to be caused by tension applied by multiple motor proteins bound to the cargo. All of the nanorods that were analyzed and discussed in the rest of the paper showed the linear directional transport without noticeable cargo rotations. Paused nanocargos undergoing restricted rotations During the axonal transport, the cargo can be in two stages: the directional (anterograde or retrograde) transport driven by the motor proteins kinesin and dynein, and the pausing stage, in which the cargo shows little or no directional movement. The pause durations vary from tens of milliseconds to tens of seconds. The cargo undergoes different motions depending on the binding status of the motor proteins to the cargo and the microtubules. The first type of motion at the pausing stage is demonstrated in Supplementary Movie 2 , in which a nanorod paused for ~6.2 s before it reversed its moving direction. The corresponding bright and dark DIC intensities of the nanorod during the whole pause period are displayed in Fig. 1a . The significant DIC intensity fluctuations indicate the fast rotational motion of the cargo during this long pause. To the best of our knowledge, this type of rotational motion has not been visualized in living cells by any other imaging techniques. 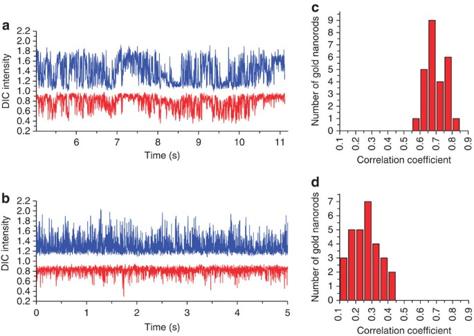Figure 1: Rotational patterns of cargos at pause and during free diffusion. (a) Normalized DIC intensities of a gold nanorod-containing cargo at a long pause during the axonal transport. The bright and dark intensities are shown in blue and red, respectively. Thex-axis (time) corresponds to the recording time ofSupplementary Movie 2. Before and after this pause, the cargo took on the directional transport. (b) Normalized DIC intensities of a gold nanorod-containing cargo freely diffusing in an axon where the microtubule arrays have been destroyed by colchicine. (c) Histogram of the correlation coefficients of the intensities of the gold nanorod-containing cargos at pauses. (d) Histogram of the correlation coefficients of the intensities of the gold nanorod-containing cargos freely diffusing in axons where the microtubule arrays have been destroyed by colchicine. Figure 1: Rotational patterns of cargos at pause and during free diffusion. ( a ) Normalized DIC intensities of a gold nanorod-containing cargo at a long pause during the axonal transport. The bright and dark intensities are shown in blue and red, respectively. The x -axis (time) corresponds to the recording time of Supplementary Movie 2 . Before and after this pause, the cargo took on the directional transport. ( b ) Normalized DIC intensities of a gold nanorod-containing cargo freely diffusing in an axon where the microtubule arrays have been destroyed by colchicine. ( c ) Histogram of the correlation coefficients of the intensities of the gold nanorod-containing cargos at pauses. ( d ) Histogram of the correlation coefficients of the intensities of the gold nanorod-containing cargos freely diffusing in axons where the microtubule arrays have been destroyed by colchicine. Full size image To better understand how the nanocargo's rotational motion is affected by the motor proteins and other associated proteins, the unrestricted rotational Brownian motion was analyzed as shown in Fig. 1b . This nanorod-containing cargo diffused freely in the axon of a differentiated PC12 cell, which had been treated with colchicine to destroy the microtubules ( Supplementary Fig. S3 ) [43] . As the cargo could no longer attach to the intact microtubules, it performed random translational and rotational diffusion. The difference in these two rotational patterns is revealed by an analysis of the degree of correlation for the bright and dark intensities. The correlated bright and dark intensity changes indicate the nanorod's in-plane rotation, whereas the anticorrelated intensity changes correspond to the out-of-plane rotation (see Supplementary Fig. S4 for details). Pearson's correlation coefficient ( r ) was thus used to analyze the DIC intensity traces with a maximum value of +1 for perfectly correlated cases, a minimum value of −1 for perfectly anticorrelated case, and the value 0 for uncorrelated cases. The correlation analysis showed that the rotational motion during the long pause ( Fig. 1a ) is distinctively different from the unrestricted rotational Brownian motion ( Fig. 1b ). The correlation coefficient for the time traces during the long pause was calculated to be 0.79. The average correlation coefficient for 26 recorded long pauses that lasted for at least 3 s was 0.70±0.06 ( Fig. 1c ). Such a large correlation coefficient suggests a high proportion of the in-plane rotational component. On the contrary, the correlation coefficient for this example of rotational Brownian motion was found to be 0.11 (close to 0, uncorrelated), suggesting the random 3D rotations with roughly equal proportions of the in-plane and out-of-plane rotational components. The average correlation coefficient for 29 recorded time traces of unrestricted rotational Brownian motion ( Fig. 1d ) was 0.26±0.09. The rotation dynamics can also be characterized using the power spectral density function. By fitting the power spectral density of the intensity traces with the Lorentzian function ( Supplementary Fig. S5 ) [44] , we found that the rotation characteristic time of the in-plane rotation at the pauses (8.7–14.3 ms) is longer than that of the random Brownian motion (2.1±0.3 ms), indicating the rotation at these long pauses is slower than the Brownian motion. The in-plane rotational motion of the cargo at the long pause leads to two new findings. First, the fast rotational motion provides direct evidence that the confinement of the rotational motions of the cargos caused by the binding of kinesin and dynein motors and possibly other associated proteins have been significantly weakened and the nanorod has gained more freedom to rotate randomly during the pauses of this type. Second, the mostly in-plane rotational motion suggests that the cargo was still tethered to the microtubule track. Otherwise, if the cargo was fully detached from the microtubule track, it would perform largely unrestricted rotational Brownian motion to generate uncorrelated bright and dark DIC intensity changing patterns (similar to Fig. 1b ) at a faster speed. The restraint could come from kinesin and dynein motors or other associated proteins such as dynactin [45] , [46] . One possibility is that the motor proteins could be deactivated by regulatory molecules but still bound to both the cargo and microtubule. The other possibility is that dynactin, which provides extra docking sites on the cargos and links the cargos to cytoplasmic dynein and microtubule tracks [47] , [48] , [49] , could also tether the cargos to the microtubules, independent of the molecular motors, and also restrict the rotational motions. In either way, the observation that the cargos performed restricted rotational motions shows that they were still tethered to the microtubule tracks at the pauses. Correlation of rotation with pause duration and moving direction Supplementary Movie 3 provides a complex example of cargo's behaviours at the directional transport and pausing stages. The corresponding bright and dark DIC intensity curves and the nanorod's lateral displacement are displayed in Fig. 2 . The nanorod-containing vesicle was transported for a distance of 4 μm retrogradely by dynein motors at ~1.0 μm s −1 in the time window of 1–5 s, paused for 5 s, and then moved again in the opposite direction by kinesin motors at a lower velocity of ~0.3 μm s −1 until the end of the recording. During both directional transport segments, the nanorod generated rather constant DIC intensities with noise expected from the DIC intensity measurements at the fast temporal resolution of 2 ms. The speed of cargo transport varied quite dramatically even in the same directional transport event as revealed by different slopes of the displacement curve. For example, the transport in Fig. 2c is much faster than that in Fig. 2d . 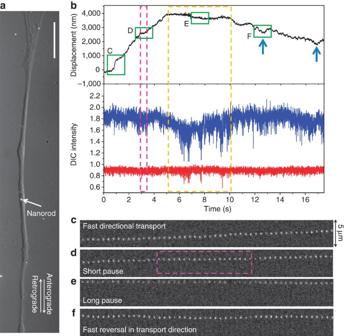Figure 2: Directional transport and pause of cargo in the axon. (a) DIC image of an axon of a differentiated PC 12 cell. A transferrin-modified gold nanorod is marked by the white arrow. The scale bar represents 10 μm. (b) Lateral displacement and normalized DIC intensities of a gold nanorod-containing cargo that was transported retrogradely, then paused, and was finally transported retrogradely again. The long pause is identified in the yellow frame, and a short pause in the pink frame. The fast reversals are highlighted by the blue arrows. (c–f) Fifty images taken fromSupplementary Movie 3at a time interval of 30 ms for each of the four regions highlighted in the green frames in (b), including (c) fast retrograde transport, (d) short pause without rotation, (e) long pause with rotation and (f) fast reversal. Figure 2: Directional transport and pause of cargo in the axon. ( a ) DIC image of an axon of a differentiated PC 12 cell. A transferrin-modified gold nanorod is marked by the white arrow. The scale bar represents 10 μm. ( b ) Lateral displacement and normalized DIC intensities of a gold nanorod-containing cargo that was transported retrogradely, then paused, and was finally transported retrogradely again. The long pause is identified in the yellow frame, and a short pause in the pink frame. The fast reversals are highlighted by the blue arrows. ( c–f ) Fifty images taken from Supplementary Movie 3 at a time interval of 30 ms for each of the four regions highlighted in the green frames in ( b ), including ( c ) fast retrograde transport, ( d ) short pause without rotation, ( e ) long pause with rotation and ( f ) fast reversal. Full size image When the cargo showed rotational motion during the 5-s pause, the bright and dark DIC intensities display a similar level of correlation ( r =0.68) as the example shown in Fig. 1a . In addition to this long pause, there were shorter pauses that lasted for tens to hundreds of milliseconds. Owing to these short pauses and other random motions, the displacement curve is far from smooth, suggesting a number of probable factors, including the competition between kinesin and dynein motors and the steric hindrance, affect the transport process continuously and result in the stochastic nature of cargo transport. The short pauses were accompanied by different cargo movement. The pink boxes in Fig. 2b and d highlight a 0.5-s pause with almost no changes in the DIC intensities, suggesting that the cargo came to a full stop without apparent rotational motion. After the pause the cargo continued to move in the same direction. The blue arrows in Fig. 2b point out another type of short pause characterized by fast reversal in the transport direction (back-and-forth movement). Many pauses of different durations were recorded. More examples are shown in Supplementary Figs S6–S9 . A statistical analysis was carried out to find the correlation between the pause duration, the rotational motion and the subsequent transport direction. For the pauses that incorporated no rotational information, the time was generally short ( Fig. 3a ), and 61 out of the 93 recorded pauses (65.6%) ended with the cargos moving in the same direction. During this type of pauses, the tension applied by motor proteins likely remained high and balanced to keep the cargos from rotating freely. The time required to resume active directional transport was generally short, and the cargos tended to maintain the original transport direction. 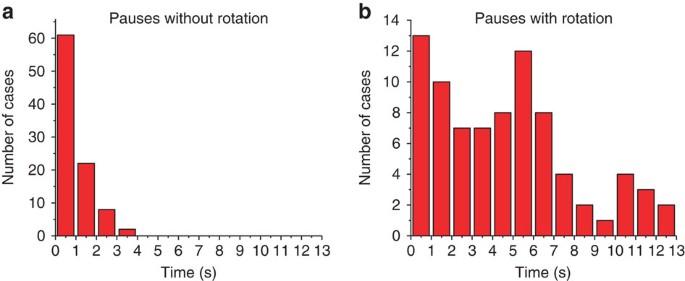Figure 3: Correlation of rotational motion at pauses with pause duration. (a) Histograms of the pause durations for 93 pauses with no apparent rotational motion. (b) Histograms of the pause durations for 81 pauses with rotational motion. Figure 3: Correlation of rotational motion at pauses with pause duration. ( a ) Histograms of the pause durations for 93 pauses with no apparent rotational motion. ( b ) Histograms of the pause durations for 81 pauses with rotational motion. Full size image For the pauses with rotation, the pause durations were generally longer with a second maximum at 5–6 s ( Fig. 3b ). During this type of pauses, the tension exerted by the motors was weakened due to the uncoupling of some motors. It is plausible that the pauses caused by the extensive uncoupling and reattachment of motors required a longer time to return to the active directional transport stage. Another important finding is that the majority of the pauses with rotation (76%, 62 out of 81 cases) were followed by the cargo transport in the reversed direction. Such a significant bias in favour of the reversed transport direction after pause indicates that the bidirectional transport of cargos should be affected by some regulatory mechanisms, instead of working in a simple unregulated stochastic manner [31] . The regulations could result in the change of single motor parameters, as the cargo transport is highly sensitive to the change of motor properties induced by regulatory mechanisms [17] . Other than the regulatory mechanisms, the long pauses observed with high occurrence of rotational motions and reversals could also be possibly due to obstacles that impede the cargos from moving forward smoothly. The unbinding and binding of the motors when confronted with an obstacle could result in extended pauses and also involve the rotational motions of the cargos. Future work to correlate these new experimental observations with computational models of motor proteins may eventually lead to a complete understanding of the complicated mechanisms. Cargo motions at track-switching Track-switching is an important consequence of pause during axonal transport. Kinesin and dynein motors frequently encounter obstacles, such as other cargos, microtubule-associated proteins, and intersecting microtubules, which obstruct their way in the transport direction [41] , [50] , [51] , [52] , [53] , [54] , [55] . The motors may pause until the track becomes available again to continue the transport, or they may overcome these obstacles by switching to other microtubules. Using SPORT, the cargo's motions during the track-switching processes were elucidated in detail. 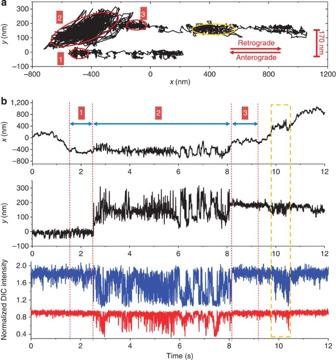Figure 4: Motions of cargo at track-switching. (a) The 2D trajectory that starts at the origin. (b) Thexandytrajectories and the normalized DIC intensity traces. The bright and dark intensities are shown in blue and red, respectively. The three steps are labelled with numbers. Another short pause with rotational motion is highlighted in the yellow frame. Figure 4a and Supplementary Movie 4 show the moving trace of a gold nanorod-containing vesicle that switched to another microtubule and reversed its moving direction after a pause. The lateral displacements in both x and y directions and the corresponding DIC intensities are shown in Fig. 4b . Three steps were visualized and identified for this track-switching process. The cargo was initially transported anterogradely by kinesin. Step 1 was a short pause with no apparent rotational motion. The nanorod moved to a new location ~100 nm away from the original location in only 2–3 frames (4–6 ms) at ~2.5 s, and started the rotation and random translational movement within a 400×200 nm region in Step 2 until ~8.1 s. In Step 3, the cargo stopped the rotational motion for ~1 s before it finally started the retrograde transport along another microtubule that was 170 nm away from the original one. The correlation coefficients of the bright and dark DIC intensities in Step 2 was 0.75, suggesting that the cargo was still tethered to the microtubule tracks and underwent the in-plane rotation. Figure 4: Motions of cargo at track-switching. ( a ) The 2D trajectory that starts at the origin. ( b ) The x and y trajectories and the normalized DIC intensity traces. The bright and dark intensities are shown in blue and red, respectively. The three steps are labelled with numbers. Another short pause with rotational motion is highlighted in the yellow frame. Full size image Apparently, the cargo 'strode' from one microtubule to another and reversed the moving direction. On the basis of the distance between the two microtubule tracks, the rotational behavior of the gold nanorod and its positions during this process, the cargo possibly went through the following steps to switch the microtubule track and reverse the moving direction. In Step 1, the cargo encountered an obstacle and stopped proceeding. In Step 2, some motors were detached from the microtubule track to give enough freedom to the cargo to rotate and swing away from the original track; in the meantime, the detached motor proteins or newly recruited ones attempted to bind to other neighbouring tracks. This was the time when both rotational and translational movements were observed in Step 2. The cargo was always tethered to the microtubules to result in the mostly in-plane rotational motion. Then, the rotational and translational movements stopped in Step 3 when enough kinesin and dynein motors and possibly other associated proteins were bound to the microtubules to prohibit the cargos from moving. At last, at the end of Step 3, the active retrograde transport was finally initiated by the dynein motors on a microtubule that was ~170 nm away from the original one. Additional examples of gold nanorods switching tracks can be found in Supplementary Figs S10 and S11 . In both examples, the cargos showed rotational behavior during the pauses before switching tracks. This can be attributed to the requirement of cargo getting loose from the original microtubule and being attached to a different one. In summary, the SPORT technique with a temporal resolution of 2 ms has been developed and used to study the axonal transport of membranous cargos. The behaviors of gold nanorod-containing cargos in both active transport and pausing stages have been elucidated in unprecedented detail. During the active transport, multiple motor proteins bind to the cargo to provide a sufficient tension to maintain the cargo's orientation. Between the active directional transport stages, the cargo experiences long and short pauses and undergoes different motions dependant upon the binding status of the kinesin and dynein motors together with other possible associated proteins such as dynactin to the cargo and the microtubule. The pauses sometimes are followed by the cargo switching to a different microtubule track. These first-time observations on the rotational dynamics of the cargo by the SPORT technique reveal how motor proteins and other associated proteins take the cargo through the alternating stages of active directional transport and pause. As a future direction, the high-speed SPORT technique will provide new evidence for understanding the mechanism of the differential modulation of kinesin and dynein motor proteins by regulating factors, such as the microtubule-associated protein tau [56] , [57] , [58] . The combination of SPORT and fluorescence microscopy will be able to correlate the rotational dynamics of cargo with interactions between motor proteins and fluorescence-labelled microtubule-associated proteins. Cell culture PC12 cells (CRL 1721. 1, ATCC, Manassas, VA) were cultured on 22×22 mm poly- L -lysine-coated coverslips in six-well cell-culturing plates. The complete cell culture medium was composed of F12K cell-culturing medium (ATCC), 15% horse bovine serum (ATCC) and 2.5% Fetal Bovine Serum (ATCC) and was added to the plates. After the cells covered 70% of the coverslips, F12 K medium supplemented with 200 ng ml −1 2.5S neuron growth factor (NGF) (Bioproducts for Science, Madison, WI, USA) was added to the plates. The cells were incubated in 37 °C incubator with 5% CO 2 for 48 h. The cell-culturing medium was then changed to F12 K medium supplemented with 200 ng ml −1 NGF and 0.05 mM forskolin (Catalog 344270, CalBiochem/EMD Biosciences). Rapid neurite extension was observed within 20 min. The differentiated PC12 cells were left in the incubator for another 48 h before use to allow the growth of intact microtubules in the axons. Preparation of transferrin-modified gold nanorods To facilitate their internalization into PC12 cells, the gold nanorods were modified with transferrin. Cetyltrimethylammonium bromide-capped (25×73 nm, 1.3×10 11 particles ml −1 , Nanopartz) gold nanorods were used. An N -hydroxylsuccinimide-PEG (NHS-PEG) disulfide linker (Sigma-Aldrich) was used by following a published protocol [59] . The NHS-PEG disulphide linker has both disulphide and succinimidyl functionalities for respective chemisorption onto gold and facile covalent coupling of transferrin molecules. Briefly, excessive surfactant was first removed from 1.0 ml of gold nanorod solution by centrifugation at 3000 g for 10 min and the particles were resuspended in 1.0 ml of 2 mM borate buffer. A proper amount of fresh NHS-PEG disulphide solution (in dimethyl sulfoxide) was added to reach a final thiol concentration of 0.2 mM and reacted with gold nanorods for 2 h. The solution was then cleaned up by centrifugation and resuspended in 2 mM borate buffer. Two microgram of transferrin was added to the gold colloidal solution and allowed to react for 8 h. Before use, the colloidal gold nanorod probes were cleaned up by centrifugation and resuspended in 2 mM borate buffer. The concentrated gold colloidal solution was diluted to a final concentration of 4.3×10 9 particles ml −1 for incubation with cells. Live-cell imaging Forty microlitre of diluted transferrin-modified gold nanorod solution were added to the cell cultures and incubated for 45 min. The coverslip was rinsed with PBS buffer (10 mM, pH 7.4) and then placed on a clean glass slide for observation. Two pieces of double-sided tape served as spacers between the glass slide and the coverslip to form a chamber. Thirty microlitre of fresh complete cell-culturing medium was added to the chamber. An upright Nikon Eclipse 80i microscope with a pair of Nomarski prisms and two polarizers was used for the imaging. The microscope was equipped with a 100×1.40 numerical aperture Plan Apo oil immersion objective and a 1.4 numerical aperture oil immersion condenser. A 700-nm optical filter (Semrock, Rochester, NY, USA) with a bandwidth of 20 nm was inserted at the illumination side. The movies were taken by a Hamamatsu ORCA-Flash2.8 CMOS camera at 500 frames s −1 . The collected videos were analyzed with MATLAB and NIH ImageJ. Microtubule destruction and fluorescence immunostaining The cells were incubated with transferrin-modified gold nanorods for 45 min and then in the cell-culturing medium containing 200 μg ml −1 colchicine for 1 h in the incubator (37 °C, 5% CO 2 ). The effect of colchicine on the microtubule network was confirmed by fixing both the treated and untreated cells with 4% paraldehyde in PBS solution and staining with the first antibody (mouse anti-alpha tubulin) and the second antibody (Alexa 488 goat anti-mouse). The fluorescent images of the destroyed microtubules after treated with colchicine and the intact microtubules in the untreated cells were observed under the Nikon Eclipse 80i microscope. Transmission electron microscopy of gold nanorod-containing vesicles The PC12 cells were plated on 22×22-mm coverslips in 3.5-cm petri-dishes and incubated with the complete cell culture medium until the cells reached over 90% confluency on the coverslips. The transferrin-modified gold nanorod solution were added into the petri-dishes to reach a final concentration of 3.7×10 10 nanoparticles per ml and the cells were incubated with the nanoparticles for 50 min at 37 °C in a cell incubator. After that, the cells were removed from the cell-culturing medium and incubated with the fixative solution containing 2.0% glutaraldehyde and 2.0% paraformaldehyde for 15 min and kept in a 4 °C fridge overnight. The cells were then postfixed with 1% osmium tetroxide in pH 7.2 PBS buffer for 1.5 h, and dehydrated in ethanol solutions with increasing concentrations of ethanol (ethanol/water v/v: 50, 60, 70, 80, 90 and 100%) for 15 min each and stained with 2% uranyl acetate in 70% ethanol solution at room temperature overnight. After that, the cells were washed three times with acetone and embedded in Epon resin. The embedded samples were removed from the coverslips and sectioned into 100 nm thick slices on a sliding ultramicrotome. The thin slices supported on the copper grids were examined with a JEOL 1200EX transmission electron microscope. Data analysis A MATLAB script was written to track the location and the DIC intensities of the gold nanorods. The constant image patterns of the gold nanorod during the directional transport facilitate the precise localization of the gold nanorods when being transported. The nanorods were localized by looking for the centre of the images. However, at the pauses when rotations occurred, the varying DIC image patterns reduced the localization precision. The actual localization precision in each image frame varies depending on the nanorod's orientation at that moment as different orientations give rise to different bright and dark DIC intensities and thus different signal-to-noise ratios. The small pixel size of the Hamamatsu CMOS camera (3.63×3.63 μm) allows the localization of gold nanorod to a precision of about 1–2 pixels or 45–90 nm. The rotation modes of the nano-cargo during the pauses were determined by calculating the Pearson's correlation coefficient of the bright and dark part intensities of the DIC images. Pearson's correlation coefficient is defined as the covariance of the two variables divided by the product of their s.d. It should be noted that the correlation coefficients were only calculated for the periods when the nanocargoes underwent rotational motions. When a nanocargo showed no apparent rotational motion, the noise would strongly affect the correlation analysis to result in mostly uncorrelated (close to 0) correlation coefficients. How to cite this article: Gu, Y. et al . Rotational dynamics of cargos at pauses during axonal transport. Nat. Commun. 3:1030 doi: 10.1038/ncomms2037 (2012).